Emergence of charge order from the vortex state of a high-temperature superconductor Evidence is mounting that charge order competes with superconductivity in high T c cuprates. Whether this has any relationship to the pairing mechanism is unknown as neither the universality of the competition nor its microscopic nature has been established. Here, we show using nuclear magnetic resonance that charge order in YBa 2 Cu 3 O y has maximum strength inside the superconducting dome, similar to compounds of the La 2− x (Sr,Ba) x CuO 4 family. In YBa 2 Cu 3 O y , this occurs at doping levels of p =0.11–0.12. We further show that the overlap of halos of incipient charge order around vortex cores, similar to those visualised in Bi 2 Sr 2 CaCu 2 O 8+ δ , can explain the threshold magnetic field at which long-range charge order emerges. These results reveal universal features of a competition in which charge order and superconductivity appear as joint instabilities of the same normal state, whose relative balance can be field-tuned in the vortex state. The enhancement of spin-stripe order by a magnetic field in La 2− x Sr x CuO 4 (ref. 1 ) and the enhanced modulation of the local density of states (LDOS) around the vortex cores in Bi 2 Sr 2 CaCu 2 O 8+ δ (Bi-2212) (ref. 2 ) are milestone results that have promoted the idea of electronic ordering that competes with superconductivity [3] , [4] , [5] , [6] , [7] . Recently, the discovery of charge order in YBa 2 Cu 3 O y appearing only for fields perpendicular to the copper-oxide planes sufficiently strong to be detrimental to superconductivity [8] , as well as the subsequent observation of related charge density wave (CDW) correlations [9] , [10] , [11] , has provided further evidence of competition. The unambiguous observation of charge order, without spin order, in this compound with a low level of disorder is significant as it reveals the ubiquity of charge-ordering tendencies in the normal state of cuprate superconductors. Furthermore, it gives unprecedented opportunities to follow, specifically by NMR, how charge order arises and develops starting deep in the superconducting state where transport techniques are inoperative, through the vortex-melting field, H melt where ultrasound measurements are blurred, up to field values comparable to H c2 , which have so far been out of reach for scattering and tunnelling techniques. Here, we show with NMR that charge order, that is, a static, long-range, spatial modulation of the charge density, emerges above a threshold magnetic field in the vortex-solid state and we show how this result can be related to earlier evidence of competing orders, thereby highlighting universal aspects of the competition between superconducting and charge orders in cuprates. These results constrain theories relating cuprate superconductivity to the charge instability. Field dependence of charge order Charge order in YBa 2 Cu 3 O y modifies the NMR lineshapes of some of the copper and oxygen ( 63 Cu and 17 O) sites in CuO 2 planes [8] ( Fig. 1 ). Here, we adopt the simplest description of these modifications, namely a line splitting [8] . Should the actual lineshape in the charge-ordered state be more complex than a simple splitting, this would affect the discussion of the exact pattern of charge order, but not the conclusions of this article, which are independent of such details. The spectral modifications induced by the charge order are relatively small, so that detecting a possible departure from a splitting or hypothetical field-dependent modifications (for instance, due to a field-dependent ordering wave-vector) is currently beyond our experimental resolution. 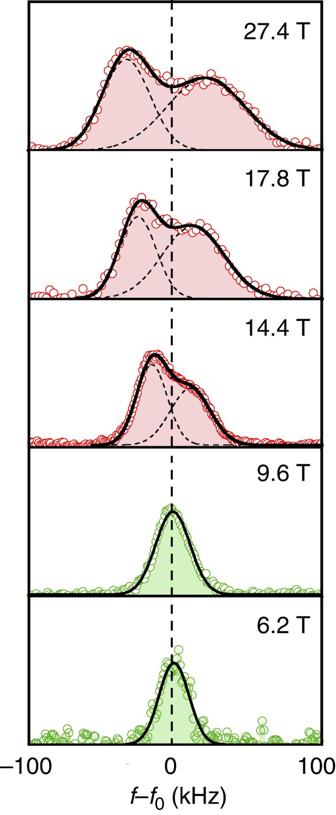Figure 1:17O NMR evidence of charge order in YBa2Cu3O6.56. Magnetic field-induced modifications of the highest-frequency quadrupole satellite of O(2) sites (lying in bonds oriented along theaaxis) atT=2.9 K and doping levelp=0.109.f0(~40–160 MHz) is the frequency of the centre of the shown spectrum. Continuous lines are fits with one Gaussian function at 6.2 and 9.6 T and with two Gaussian functions (each shown as a dotted line) at higher fields. See Methods section for more information about the17O spectra. Figure 1: 17 O NMR evidence of charge order in YBa 2 Cu 3 O 6.56 . Magnetic field-induced modifications of the highest-frequency quadrupole satellite of O(2) sites (lying in bonds oriented along the a axis) at T =2.9 K and doping level p =0.109. f 0 (~40–160 MHz) is the frequency of the centre of the shown spectrum. Continuous lines are fits with one Gaussian function at 6.2 and 9.6 T and with two Gaussian functions (each shown as a dotted line) at higher fields. See Methods section for more information about the 17 O spectra. Full size image The net line splitting involves a splitting Δ ν magn of magnetic hyperfine origin and a splitting Δ ν quad of electric quadrupole origin. As ν quad at Cu and O sites in the cuprates is a linear function of p (ref. 12 ), we take Δ ν quad to be, in the first approximation, a measure of a charge density difference, that is, the amplitude of the charge order. The expression ‘charge order’ will be used here generically, with no regard given to its specific morphology, such as, uni- or bi-directional, or its microscopic origin such as Fermi surface instability, electron–phonon coupling or strong correlation effect. The sharp temperature dependence of the NMR splitting below the onset temperature T charge (ref. 6 ) ( Fig. 2a ) and recent ultrasound measurements [13] already indicate that charge order occurs through a phase transition. However, up to now, the field dependence for T << T charge has not been accessed. The new central result is our observation at T ≈3 K of a sharp square-root-type increase of Δ ν quad , Δ ν quad ( H−H charge ) 1/2 , starting above a threshold field, H charge ≈10.4 T in a sample having p =0.109 and ortho-II oxygen order ( Fig. 3a ). Qualitatively similar results, albeit covering a smaller field range, were obtained for three other samples from either 63 Cu or 17 O NMR ( Fig. 3b-d ). This constitutes the first example of a (apparently second order) quantum phase transition, controlled by the magnetic field, from a homogeneous d -wave superconductor to a superconductor with charge order. Remarkably, the low values of the magnetic hyperfine shift K at low T ( Fig. 2c ) reveal a vanishing of the spin susceptibility, which persists in high fields. Charge ordering thus leaves the pseudogap intact. 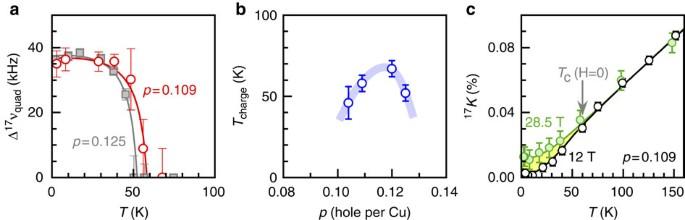Figure 2: Temperature-induced transition towards charge order in the pseudogap state. (a) Quadrupole part of the splitting of the highest-frequency O(2) quadrupole satellite forp=0.109 andp=0.125 (see Methods for details) as a function of temperature in fields of 27.4 and 28.8 T, respectively. The lines are guides to the eye. (b) Transition temperatureTchargeshowing a maximum around hole-dopingp=0.115–0.12. The thick trace is a guide to the eye. (c) Magnetic hyperfine shift17Kof O(2,3) sites forp=0.109 andH||c. No anomalous change of17Kis observed acrossTcharge. At low temperature in the charge-ordered state, the maximum shift variation Δ17K≈0.01% between 12 and 28.5 T (yellow region) represents a minor change compared to the decrease Δ17K≈0.12% betweenT=300 K and 60 K associated with the pseudogap42. The pseudogap is thus essentially unaffected by the occurrence of charge order. This result agrees with the relatively modest size of the field-induced changes in the63Cu relaxation rate 1/T1(ref.8). The field dependence of17KbelowTcarises from the density of nodal states in ad-wave superconductor43. Error bars represent s.d of the fit parameters. Figure 2: Temperature-induced transition towards charge order in the pseudogap state. ( a ) Quadrupole part of the splitting of the highest-frequency O(2) quadrupole satellite for p =0.109 and p =0.125 (see Methods for details) as a function of temperature in fields of 27.4 and 28.8 T, respectively. The lines are guides to the eye. ( b ) Transition temperature T charge showing a maximum around hole-doping p =0.115–0.12. The thick trace is a guide to the eye. ( c ) Magnetic hyperfine shift 17 K of O(2,3) sites for p =0.109 and H || c . No anomalous change of 17 K is observed across T charge . At low temperature in the charge-ordered state, the maximum shift variation Δ 17 K ≈0.01% between 12 and 28.5 T (yellow region) represents a minor change compared to the decrease Δ 17 K ≈0.12% between T =300 K and 60 K associated with the pseudogap [42] . The pseudogap is thus essentially unaffected by the occurrence of charge order. This result agrees with the relatively modest size of the field-induced changes in the 63 Cu relaxation rate 1/ T 1 (ref. 8 ). The field dependence of 17 K below T c arises from the density of nodal states in a d -wave superconductor [43] . Error bars represent s.d of the fit parameters. 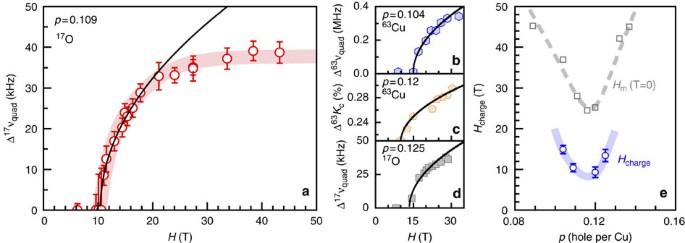Figure 3: Quantum phase transition to the charge-ordered state. (a) Quadrupole part of the splitting of the O(2) line shown inFig. 1forp=0.109 andT≈3 K (see Methods for details). The thick red trace is a guide to the eye. The thin black line is a fit to (H−Hc)0.5. (b) Quadrupole splitting of63Cu(2F) (planar Cu sites below oxygen-filled chains) forp=0.104 (ortho-II) atT=2 K. (c) Full linewidth at half maximum of the63Cu central line forp=0.12 (ortho-VIII) atT=1.4 K. Because of the broad and complex Cu spectra in this sample, the splitting of the63Cu satellite line could not be observed8. However, the width of the central line reflects the modifications of the lineshape due to charge order modulating the hyperfine fields8. (d) Quadrupole part of the splitting of the17O(2) line forp=0.125 (ortho-VIII) atT=2.1 K. (e) Hole-doping dependence of the onset fieldHchargeas determined from a fit of the data to (H−Hcharge)0.5(thin black lines ina–d). The minimum ofHchargenearp=0.115–0.12 parallels that of the vortex-melting fieldHmelt(T→0), which has been argued to reflect the upper critical fieldHc2(T→0) (ref.15). Error bars represent s.d. in the fit parameters. Full size image Figure 3: Quantum phase transition to the charge-ordered state. ( a ) Quadrupole part of the splitting of the O(2) line shown in Fig. 1 for p =0.109 and T ≈3 K (see Methods for details). The thick red trace is a guide to the eye. The thin black line is a fit to ( H − H c ) 0.5 . ( b ) Quadrupole splitting of 63 Cu(2F) (planar Cu sites below oxygen-filled chains) for p =0.104 (ortho-II) at T =2 K. ( c ) Full linewidth at half maximum of the 63 Cu central line for p =0.12 (ortho-VIII) at T =1.4 K. Because of the broad and complex Cu spectra in this sample, the splitting of the 63 Cu satellite line could not be observed [8] . However, the width of the central line reflects the modifications of the lineshape due to charge order modulating the hyperfine fields [8] . ( d ) Quadrupole part of the splitting of the 17 O(2) line for p =0.125 (ortho-VIII) at T =2.1 K. ( e ) Hole-doping dependence of the onset field H charge as determined from a fit of the data to ( H−H charge ) 0.5 (thin black lines in a – d ). The minimum of H charge near p =0.115–0.12 parallels that of the vortex-melting field H melt (T→0), which has been argued to reflect the upper critical field H c2 (T→0) (ref. 15 ). Error bars represent s.d. in the fit parameters. Full size image Relationship with other probes of charge order in YBa 2 Cu 3 O y The finite value of H charge suggests that there is no static long-range charge order in zero field, in agreement with the interpretation of X-ray results in terms of CDW fluctuations [9] . We note that our H charge ≈9.3 T for p =0.12 corresponds approximately to the field above which the intensity and the width of the superlattice peaks in X-ray measurements [10] become larger in the low-temperature limit ( T =2 K) than at 66 K, that is at the zero-field T c . This suggests that H charge corresponds to a threshold in the screening of the CDW correlations by the superconducting regions of the sample (see next section for a more precise interpretation of this threshold). On the other hand, sound velocity data [13] for p =0.108 suggest H charge ≈18 T ( c 11 mode) and H charge ≈16±2 T (other modes), both larger than H charge ≈10.4±1.0 T in NMR for p =0.109. It is possible that NMR somewhat underestimates H charge if pre-transitional effects modify the lineshape below the real H charge . This should lead to some caution regarding the precise value of H charge but it does not affect the conclusions of this paper. Relationship with vortex physics For all samples, H charge ≈9–15 T is found to be lower than the melting transition of the vortex lattice that takes place at H melt >20 T for T ≤5 K (ref. 14 ). The charge-ordering transition thus occurs inside the vortex-solid phase. As the vortex cores represent normal regions of radius ξ SC within the superconductor, it is expected [15] , [16] , [17] that the charge fluctuations detected above T c (refs 9 , 10 , 11 ) continue to develop at low temperatures within the cores where they escape the competition with superconductivity. As suggested by LDOS modulations in Bi-2212 (ref. 2 ), halos of incipient charge order are centred on the cores and they extend over a typical distance ξ charge > ξ SC ( Fig. 4 ). On increasing the field, the long-range, static, charge order may be expected to appear when these halos start to overlap. This should occur at H charge = Φ 0 /(2 πξ charge [2] ), as the halo density equals the density of vortices whose cores start to overlap at the upper critical field, H c2 = Φ 0 /(2 πξ SC 2 ). Owing to our observation of a field-induced transition to the charge-ordered state, this prediction is now confirmed by experiments for the first time: H charge =9.3±1.3 T for p =0.12 (ortho-VIII) translates into ξ charge =16 a , where a is the planar Cu–Cu distance. This is to be compared to ξ charge ≈19 a measured at H =9 T and T =2 K by X-ray diffraction for the same doping level [10] . Despite the obvious simplistic nature of the description (for instance, neither a coupling between CuO 2 planes nor an in-plane anisotropy of ξ charge is considered), this agreement suggests that this picture is indeed the correct starting point for explaining the field-induced transition. This is the second central result of this work. 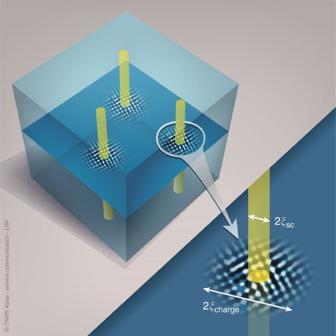Figure 4: Halos of incipient charge order centred on vortex cores. The yellow tubes represent the vortex cores of radius given by the superconducting coherence lengthξSC. Black and white halos represents sites with high and low charge density. The actual pattern of the charge density modulation has no role in the discussion of this paper, so its schematic representation is arbitrary here. Such halos of incipient charge order start to overlap atHchargeand thus induce long-range order. This description, inspired from scanning tunnelling microscopy results in Bi-2212 (ref.2), is quantitatively consistent with our results in YBa2Cu3Oy(see text).ξchargeis the typical length over which the charge density is correlated, thus defining halos of diameter 2ξchargearound the vortex cores (image used with permission; CNRS Alpes—service communication—LRF). Figure 4: Halos of incipient charge order centred on vortex cores. The yellow tubes represent the vortex cores of radius given by the superconducting coherence length ξ SC . Black and white halos represents sites with high and low charge density. The actual pattern of the charge density modulation has no role in the discussion of this paper, so its schematic representation is arbitrary here. Such halos of incipient charge order start to overlap at H charge and thus induce long-range order. This description, inspired from scanning tunnelling microscopy results in Bi-2212 (ref. 2 ), is quantitatively consistent with our results in YBa 2 Cu 3 O y (see text). ξ charge is the typical length over which the charge density is correlated, thus defining halos of diameter 2 ξ charge around the vortex cores (image used with permission; CNRS Alpes—service communication—LRF). Full size image Doping dependence of charge order around p =0.11–0.12 On increasing the field further in the p =0.109 sample, Δ ν quad saturates at fields of 30–35 T ( Fig. 3a ). Remarkably, this field scale is similar to H c2 , as defined from transport measurements in these samples [14] , [18] , [19] , [20] , indicating that the growth of the amplitude of the charge order is controlled by the decrease of the superconducting order parameter. Although the precise value of H c2 is a matter of debate [21] , a dip of H c2 near p =0.115–0.12 and values in the range 24–60 T appear to be robust conclusions. Furthermore, this dip of H c2 is paralleled by both a minimum of H charge ( Fig. 3e ) and by a maximum of T charge near p =0.115–0.12 ( Fig. 2b ). These correlations are again a manifestation of the competition between superconductivity and charge order and they are consistent with charge order being strongest near p =0.115–0.12 (ref. 22 ), which is within the superconducting dome. This last observation is, however, puzzling. On one hand, there is an obvious parallel with the stabilisation of charge stripes of period λ ≈4 a at a similar (but not strictly identical) doping of p =0.125=1/8 in compounds of the La-214 family such as La 2− x Ba x CuO 4 and possibly in Bi-2212 as well [23] . This similarity would be natural if the CDW in YBa 2 Cu 3 O y ( p ≈0.12) also had λ ≈4 a . On the other hand, if the charge order is incommensurate with λ ≈3.3 a (refs 9 , 10 , 11 ), there is no obvious reason why it should be more stable near p ≈0.12, especially because the chain-oxygen order does not seem to have a prominent role in determining H charge given our finding of similar H charge values in ortho-II ( p =0.109) and ortho-VIII ( p =0.12) samples ( Fig. 3e ). Even if our understanding of the charge order in YBa 2 Cu 3 O y (and perhaps of the 1/8 problem in general) is incomplete, the results reported here reveal an outstanding universality of magnetic field effects in underdoped cuprates. Indeed, a competition between superconductivity and charge order has also been argued [6] , [15] , [16] , [17] to provide a natural explanation of the field-enhanced spin and charge orders in La-214 (refs 1 , 3 , 4 , 5 , 6 ) and LDOS modulations in Bi-2212 (refs 2 , 7 ). Despite possible differences in the morphology of the charge order that may depend on the crystallographic structures and on the level of disorder in different families of cuprates, the above experiments and the results in YBa 2 Cu 3 O y are all consistent with the idea that a magnetic field applied perpendicular to the CuO 2 planes generates vortices around which fluctuating or weakly pinned, short-range charge order is revitalised. The long-range order that should follow from the charge instability of the normal state is initially hindered by superconductivity, but it eventually sets in when a sufficiently high density of vortices is reached. On the other hand, when charge order and superconductivity already coexist in zero field, the charge order is simply enhanced by the field [6] . This field-tuned competition differs from the simple coexistence of CDW order and superconductivity in, for example, NbSe 2 for which the onset of superconductivity occurs well below the CDW transition and does not affect CDW order. Therefore, the magnetic field has no effect on the CDW [24] . The competition in cuprates is apparently also different from the coexistence of two adjacent phases in the phase diagram of other unconventional superconductors: in this case, the transition to the competing phase can take place at a much higher temperature than superconductivity, which occurs near the verge of this competing phase [25] . Here, in contrast, the maximum of T charge (and H charge ) occurs at p =0.11–0.12 within the superconducting dome and the transition temperatures are similar ( T c ~ T charge ), indicating that the two orders have very close energy scales near p =0.11–0.12. Such near-degeneracy suggests that, although competing, charge order and superconductivity are joint instabilities of the same normal (pseudogap) state in this doping range. Despite the mounting evidence for a charge-ordering instability in virtually all cuprate families [2] , [6] , [8] , [9] , [10] , [11] , [23] , [26] , [27] , [28] , [29] , [30] , there is still a long way to go before elucidating the importance of this instability in determining the properties of the cuprates. Neither the possibility of an intertwining of the charge and superconducting order parameters [31] nor the possibility of a direct relationship between the two orders [32] , [33] can be addressed by the present results. Furthermore, more work is needed to understand whether the interplay between charge ordering and superconductivity is fundamentally, or only superficially, different from that in other systems showing CDW and superconducting orders in their phase diagrams [34] , [35] . The most pressing question for clarifying these issues is now to determine how far the charge correlations extend in the temperature versus doping phase diagram. Samples High-quality, oxygen-ordered ( Supplementary figure S1 ), detwinned single crystals of YBa 2 Cu 3 O y were grown in non-reactive BaZrO 3 crucibles from high-purity starting materials [36] . Two samples were enriched with the oxygen-17 ( 17 O) isotope that, unlike 16 O, possesses a nuclear spin. Table 1 summarises the properties of the four samples studied in this work. Note that the p -values are obtained on the basis of the values of the superconducting transition temperature T c , as measured by SQUID, using the standard calibration [37] . As this calibration was established for samples with 16 O, the isotope effect on the transition temperature T c of the 17 O-enriched samples must be taken into account. As 16 O→ 18 O exchange produces a change Δ T c ≈−2 K in the Y-123 system with T c values around 60 K (ref. 38 ), the hole content of the two 17 O-enriched crystals was estimated using a T c value corrected by Δ T c =+1 K with respect to their T c value measured by SQUID. This is based on the standard expression for the isotope effect Δ T c / T c =− α Δ M / M , where M is the isotope mass and α is the isotope effect exponent ( α ≈0.27 here in YBa 2 Cu 3 O y ). The correction for 16 O→ 17 O exchange is thus half of that for 16 O→ 18 O. Table 1 Composition and characteristics of the samples reported in this study. Full size table NMR spectra of quadrupolar nuclei The resonance frequency of a given ( m ↔ m −1) transition for a nucleus of spin I >1/2 is given by the sum of magnetic hyperfine and electric quadrupole contributions [39] : with− I +1≤ m ≤ I , v magn =(1+ K zz ) v ref , where K zz is the component of the hyperfine magnetic shift tensor along the magnetic field direction and v ref = γH is a reference frequency (such as the resonance frequency of the bare nucleus in vacuum or the resonance frequency of the nucleus in a substance without unpaired electrons). To first order in perturbation (although not negligible, the second order is not necessary for the simple qualitative background that we intend to provide here), where is the quadrupole frequency, and , where V is the electrostatic potential at the nucleus position and is the corresponding electric field gradient tensor. The principal axes ( X , Y , Z ) of the tensor are defined such that | XX |≤| YY |≤| ZZ | and the asymmetry parameter η=( XX − YY )/ ZZ . θ is the polar angle between the magnetic field direction z and ZZ and φ is the azimuthal angle in the ( x , y ) plane perpendicular to the field. For planar 63 Cu, Z is the crystalline c axis, while for planar 17 O, Z is the Cu–O–Cu direction (that is, a for O(2) and b for O(3)). Supplementary figure S2 shows a sketch of a typical quadrupole-split NMR spectrum. Understanding precisely how the charge density modulation affects the electric field gradient and thus modifies Δ ν quad = f ( ν Q , η , θ , φ ) requires complex ab initio calculations that are beyond the scope of this article. As ν quad at Cu and O sites in cuprates is a linear function of p (ref. 13 ), we take Δ ν quad to be, in the first approximation, a measure of a charge density difference, which is the amplitude of charge order. NMR methods Experiments were performed in the LNCMI-Grenoble resistive magnets M1, M9 and M10 as well as in the NHFML hybrid magnet. Standard spin-echo techniques were used with heterodyne spectrometers. Spectra were obtained at fixed magnetic fields by combining Fourier transforms of the spin-echo signal recorded for regularly spaced frequency values [40] . The 27 Al NMR reference signal from metallic aluminium was used to calibrate the external magnetic field values. The 17 K measurements were performed with H || c , on the central line, that is the (−1/2↔1/2) transition, where O(2) and O(3) sites overlap. The 17 K values thus represent average values for these two sites. Neither the very weak and broad 17 O signal from the chains nor the sharp signal from apical 17 O sites significantly affected the determination of the position of the O(2,3) central line. 17 K values are given with respect to the resonance frequency of the bare nucleus and they are in excellent agreement with earlier works [41] . In order to determine the 17 O line-splitting, the magnetic field was tilted by θ =16° off the c axis in order to separate O(2) from O(3) satellite transitions. In that case, the quoted magnetic field values correspond to the c axis component (that is they are corrected by a factor cos(16°)=0.961 with respect to the total external field values), which is justified by the disappearance of charge order when H c (ref. 8 ). We report here the field-induced modifications of the O(2) NMR lines, which are those sites from Cu–O–Cu bonds aligned along the a axis, which is perpendicular to the chain direction b . Clear field-induced spectral modifications are also observed for O(3E) and/or O(3F) sites (planar sites in bonds along b , below empty and filled chains, respectively), but these could not be easily analysed as the O(3E) and O(3F) lines overlap. A complete account and interpretation of 17 O NMR spectra in the charge-ordered state is beyond the scope of the present work and will be published separately (Wu et al ., in preparation). Analysis of NMR spectra The separation of the magnetic hyperfine, Δ ν magn , and quadrupole, Δ ν quad , contributions to the total line splitting was performed by reproducing the experimental positions of 63 Cu(2F) or 17 O(2) lines with a simulation based on an exact diagonalisation of the nuclear-spin Hamiltonian. For 17 O(2), it is also possible to extract Δ ν quad by subtracting the total splitting Δ ν total (1)=Δ ν magn +Δ ν quad of the (1/2↔3/2) satellite from the total splitting Δ ν total (2)=Δ ν magn +2Δ ν quad of the (3/2↔5/2) satellite. However, Δ ν total (1) is not always experimentally accessible. For p =0.09, the saturation of Δ ν quad and Δ ν magn above ~30 T is confirmed by the linear field dependence of the total splitting Δ ν =Δ ν quad +Δ ν magn =Δ ν quad +Δ K zz γH , and by the perfect overlap of the lineshapes of the 63 Cu central transition at all fields >30 T when plotted in a frequency scale normalised by field. No stable fit of the temperature dependence of Δ v quad could be performed close to T charge . Nevertheless, we found that the temperature dependence of the guide to the eye shown in Fig 2a for the p =0.125 data also matches very well the data for p =0.104 (ref. 8 ) and p =0.109. We thus used this guide to determine the transition temperature of the charge-ordered state, T charge . H charge is determined by fitting Δ v quad data to ( H - H charge ) 0.5 , so that the result does not depend on the points for which Δ v quad is assumed to be zero. The value of H charge is largely determined by the curvature of Δ v quad versus H : that is, the data points for which the large splitting results in relatively small error bars contribute as much as the points close to H charge , which have larger error bars. The data for the p =0.109 sample were fit to ( H − H charge ) α and the fit resulted in α =0.49±0.09. How to cite this article: Wu, T. et al . Emergence of charge order from the vortex state of a high temperature superconductor. Nat. Commun. 4:2113 doi: 10.1038/ncomms3113 (2013).